Strong ferromagnetism at the surface of an antiferromagnet caused by buried magnetic moments Carrying a large, pure spin magnetic moment of 7 μB per atom in the half-filled 4 f shell, divalent europium is an outstanding element for assembling novel magnetic devices in which a two-dimensional electron gas may be polarized due to exchange interaction with an underlying magnetically-active Eu layer. Here we show that the Si-Rh-Si surface trilayer of the antiferromagnet EuRh 2 Si 2 bears a surface state, which exhibits an unexpected and large spin splitting controllable by temperature. The splitting sets in below ~32.5 K, well above the ordering temperature of the Eu 4 f moments (~24.5 K) in the bulk, indicating a larger ordering temperature in the topmost Eu layers. The driving force for the itinerant ferromagnetism at the surface is the aforementioned exchange interaction. Such a splitting may also be induced into states of functional surface layers deposited onto the surface of EuRh 2 Si 2 or similarly ordered magnetic materials with metallic or semiconducting properties. For a long time, rare-earth (RE) intermetallic materials have attracted considerable interest because of their exotic properties at low temperatures, which include complex magnetic phases, valence fluctuations, heavy-fermion states, Kondo behaviour and many others [1] , [2] , [3] , [4] , [5] , [6] , [7] . Europium with its half-filled 4 f shell has a unique position among the lanthanides. For the free Eu atom and the Eu metal, the 4 f 7 configuration—corresponding to a divalent Eu state—is the stable one, but in many intermetallic compounds the Eu 4 f shell is occupied by six electrons only. Since both configurations are nearly degenerate in energy, tiny changes in stoichiometry, doping or external parameters like pressure and temperature may lead to transitions from a divalent [Xe]4 f 7 (5 d 6 s ) 2 to a trivalent [Xe]4 f 6 (5 d 6 s ) 3 state of Eu, or even stabilize mixed-valent behaviour. According to Hund’s rules, the 4 f 6 configuration is a Van-Vleck paramagnet with zero total effective angular momentum in the ground state, while the divalent 4 f 7 configuration reveals a large pure spin momentum ( J = S =7/2) and can give rise to sophisticated magnetic properties in Eu-based intermetallics. In this regard, EuRh 2 Si 2 is apparently well-suited to give insight into the interplay between magnetic and electronic degrees of freedom [8] . Here, Eu exhibits a stable 4 f 7 configuration (Eu 2+ ) from low temperature to room temperature with a pure spin magnetic moment of 7 μB. It crystallizes in the tetragonal body-centered ThCr 2 Si 2 structure [8] , [9] , similarly to the heavy-fermion YbRh 2 Si 2 system [10] , [11] or the famous ‘hidden order’ material URu 2 Si 2 (ref. 12 ). Its electronic structure is strongly correlated, involving massless and heavy quasiparticles, which are mutually interacting [13] . Below the Néel temperature T N =24.5 K the Eu 4 f moments in EuRh 2 Si 2 order antiferromagnetically (AFM) [8] . Like in several other RERh 2 Si 2 compounds, the magnetic structure of EuRh 2 Si 2 is composed of ferromagnetic Eu layers in the ab planes stacking AFM along the c axis. Reflections corresponding to an incommensurate propagation vector (0 0 τ ) along the c axis are clearly seen in resonant magnetic X-ray scattering at the Eu L 3 edge below T N . Here we report on strong ferromagnetic properties of the surface and subsurface region in the antiferromagnet EuRh 2 Si 2 , which are driven by the ordered local 4 f moments of Eu. These properties are monitored by angle-resolved photoelectron spectroscopy (ARPES) looking at the diamond-shaped surface state that exists around the point of the surface Brillouin zone. This Shockley-type surface state is observed at the Si-terminated surface, and resides inside a large gap in the projected bulk band structure. The surface ferromagnetism is manifested by a huge splitting of this state due to the exchange interaction with the ordered local moments of the Eu atoms lying three atomic layers below the surface. The exchange splitting of the surface state, which may be described as a trapped two-dimensional electron gas within the top four layers, provides immediate information on the magnetism of the first buried Eu layer in EuRh 2 Si 2 when followed, for instance, as a function of temperature. Moreover, this splitting can be generally used as an experimental fingerprint of surface ferromagnetism for layered materials. ARPES insight into the surface ferromagnetism In Fig. 1 we show the Fermi surface and the electron band structure for the Si-terminated surface of EuRh 2 Si 2 as seen in ARPES at low temperatures ( T =11 K). The most explicit feature here is a diamond-shaped surface state, lying inside a large gap of the projected bulk band structure around the point of the surface Brillouin zone. Like in YbRh 2 Si 2 (ref. 10 ), this Shockley-like surface state is created mainly by Si 3 s , 3 p (57%) and Rh 4 d (38%) states (the lacking 5% stem from the Eu 5 d derived states) and is intrinsic to the silicon-terminated (001) surface. However, unlike in YbRh 2 Si 2 , the surface state in EuRh 2 Si 2 reveals a clear and strong splitting. Because of this difference a Rashba-type spin–orbit interaction seems not to be the origin of the observed splitting, as it should be present in YbRh 2 Si 2 as well. A more plausible scenario of the detected splitting is a magnetic exchange interaction of the surface state with Eu 4 f moments in the first buried Eu layer below the surface. Note that an exchange type splitting of the surface state implies ordered local moments in the first Eu layer, which is in line with the observed in-plane ( ab ) ferromagnetic order ( Supplementary Fig. 1 and Supplementary Note 1 ). A related phenomenon has been reported for the helical antiferromagnet holmium [14] with the main difference that there the Ho d -states couple to the 4 f moments on the same site, while in the present case the surface state of the outermost Si-Rh-Si plane couples to Eu-moments in the fourth subsurface layer. 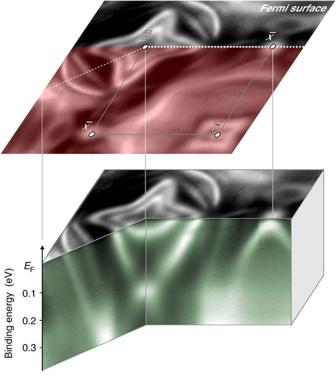Figure 1: Fermi surface and electron bands for the AFM phase of EuRh2Si2. Three-dimensional representation of the ARPES-derived electron band structure measured at 11 K for a Si-terminated surface of EuRh2Si2around thepoint of the surface Brillouin zone. Figure 1: Fermi surface and electron bands for the AFM phase of EuRh 2 Si 2 . Three-dimensional representation of the ARPES-derived electron band structure measured at 11 K for a Si-terminated surface of EuRh 2 Si 2 around the point of the surface Brillouin zone. Full size image The assignment of the surface state splitting to exchange interaction with a magnetic sublayer is supported by measurements performed on a freshly cleaved crystal at T =35 K, that is, above the Néel temperature. Indeed, no splitting of the surface state is observed at this temperature, as seen in Fig. 2a,b , where we show the experimentally observed Fermi surfaces around the point at high and low temperatures, respectively. When we follow the evolution of the surface state with decreasing temperature ( Fig. 2c ), we can see that the splitting sets in rather sharply at around 32.5 K and rapidly reaches a value of about ~150 meV ( Fig. 2d ) where it levels off. Note that the onset of the splitting is notably above the bulk ordering temperature, T N =24.5 K, indicated by the dashed line. The temperature evolution of the splitting was determined by looking at a cut parallel to, but slightly away from the high symmetry direction – ( Fig. 2d , Supplementary Fig. 2 , and Supplementary Note 2 ). The situation at the point is not suitable to study the temperature dependence of the aforementioned spin splitting, because at this point there is a strong interference of the electron-like surface state with a hole-like band leading to hybridization ( Supplementary Figs 3,4 ) and a gap formation near the point. 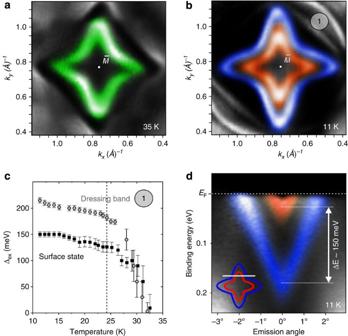Figure 2: ARPES insight into the magnetically induced split of the diamond-shaped surface state. Fermi surface maps taken for the Si-terminated surface of EuRh2Si2near thepoint at 35 K (a) and at 11 K (b), that is, above and below the bulk AFM transition atTN=24.5 K, respectively. (c) The ARPES-derived temperature evolution of the magnitude of the surface state (dark symbols) and dressing band’s (light symbols) split. For both, the split vanishes above ~32.5 K. The data points are shown with error bars. (d) The ARPES-derived band map taken at 11 K, demonstrating the largest splitting of the surface state. The inset schematically shows the direction of the measurements. Figure 2: ARPES insight into the magnetically induced split of the diamond-shaped surface state. Fermi surface maps taken for the Si-terminated surface of EuRh 2 Si 2 near the point at 35 K ( a ) and at 11 K ( b ), that is, above and below the bulk AFM transition at T N =24.5 K, respectively. ( c ) The ARPES-derived temperature evolution of the magnitude of the surface state (dark symbols) and dressing band’s (light symbols) split. For both, the split vanishes above ~32.5 K. The data points are shown with error bars. ( d ) The ARPES-derived band map taken at 11 K, demonstrating the largest splitting of the surface state. The inset schematically shows the direction of the measurements. Full size image Looking closely and comparing Fig. 2a,b , we may also detect the splitting of the ‘dressing band’, labelled as ‘1’. This splitting shows temperature dependence similar to that of the diamond-shape surface state, which is presented in Fig. 2c too, and will be discussed below. Origin of the Shockley surface state splitting If we ascribe the magnetic splitting of the surface state to exchange interactions with the localized 4 f moments of the topmost Eu layer, then the size of the splitting represents a direct measure of the magnetization of the Eu plane in the crystal. The fact that the splitting disappears only notably above the bulk Néel temperature suggests that a certain in-plane order of the Eu 4 f moments in the topmost Eu layer persists even above the bulk ordering temperature. Two scenarios could explain this phenomenon: magnetic fluctuation in the paramagnetic (PM) region or a static ferromagnetic order in the topmost Eu layer. Magnetic fluctuations, that is, domains in the PM region that reveal for short time magnetic order above the bulk ordering temperature are well-known phenomena and occur on a timescale that is usually large compared with the characteristic timescale of the photoemission process of 10 −16 s (refs 15 , 16 ). With certain probability magnetically-ordered domains could then be observed in the photoemission experiment, which may explain the experimental results and reflect predominantly a bulk magnetic property. However, the temperature dependence of the splitting, which is proportional to the magnetization, is rather reminiscent of the power-law behaviour observed close to a second-order phase transition (see Fig. 2c ). Therefore, the discussed fluctuating magnetic order scenario seems unlikely, and there are some indications for a specific magnetic phase close to the surface. The persistence of static magnetic order in the topmost Eu layer even above the bulk ordering temperature is a more likely scenario. Such an effect is known, for instance, from ferromagnetic Gd metal where ferromagnetic order in the outermost surface layer is observed up to 60–80 K above the bulk Curie temperature [17] , [18] , [19] and reveals all features of an extraordinary phase transition [20] . In Gd this phenomenon seems to be related to the existence of a weakly dispersing surface state of d z 2 -symmetry, which reveals a characteristic Stoner-like splitting that scales with the magnetization of the outermost Gd plane [19] . The Gd system thus seems to be similar to EuRh 2 Si 2 . However, in EuRh 2 Si 2 the responsible magnetic moments are not located directly at the surface but in the fourth subsurface layer and the surface state is not formed by RE derived orbitals but mainly by Si 3 s , 3 p and Rh 4 d states of the topmost Si-Rh-Si trilayer. How could, in this case, the spin polarization be transferred from the ferromagnetic subsurface Eu layer through several atomic layers into the surface state? In metallic RE compounds, magnetic order is usually mediated by an oscillatory spin polarization of conduction electrons (RKKY interaction). In this picture, the localized 4 f electrons polarize Eu 5 d states, which in turn hybridize with ligand states and transfer the spin polarization. As a free atom, divalent Eu reveals a [Xe]4 f 7 6 s 2 configuration without any electron populating the 5 d shell; in the solid, however, hybridization leads to finite 5 d occupancy that amounts in case of EuRh 2 Si 2 to ~0.84 electrons per Eu site. In bulk EuRh 2 Si 2 , the oscillatory RKKY interaction changes its sign along the c axis across a Si-Rh-Si trilayer leading to antiferromagnetic coupling of adjacent Eu layers. Therefore, while in the case of an Eu-terminated surface one expects spin polarization of the outermost Eu atoms, in the case of the present Si-terminated surface spin polarization within the outermost Si-Rh-Si trilayer is expected to be very weak. For a nearly free-electron-like band, a splitting of 150 meV would correspond to an internal field of 1,300 T. Such a huge field can only be induced by exchange. It cannot be ascribed to magnetostatic interaction with the dipole fields of the Eu 4 f moments: assuming an average distance of about 1 Å between the surface state and the outermost Eu layer, the resulting energy splitting would amount to less than 1 meV, that is, two orders of magnitude smaller than observed. Theoretical insight into the surface and bulk related magnetism To investigate the possibility of such an exchange interaction across four atomic layers we performed a density functional theory (DFT)-based analysis of the discussed experimental findings. To this end, we calculated and compared the band structures in the surface region assuming several magnetic configurations including the bulk PM and AFM phases. In Fig. 3 we present the results of respective calculations for the latter two configurations. Note here that in these calculations spin–orbit interaction was not included, however, we will discuss below how its inclusion would affect the bands of the surface state. 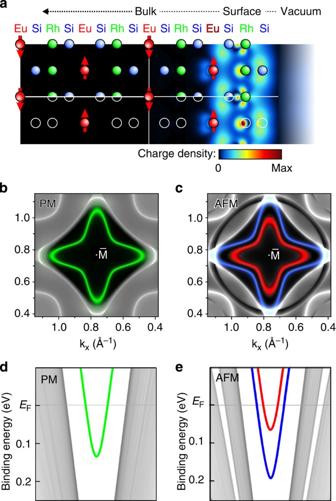Figure 3: Theoretical insight into surface and bulk related electrons in EuRh2Si2. (a) Probability density distribution (projected on theacplane) of the surface states at thepoint obtained for the PM phase, which is superimposed with the slab crystal structure used for band-structure calculations. (b,c) The computed and superimposed Fermi surfaces for bulk and slab calculations for the PM and AFM phases, respectively. Here, the diamond-shaped surface states lie in the huge gap (black) of the projected bulk bands (grey) around thepoint. For the PM and AFM phases the surface state is emphasized in green (unsplitted) and red-blue (splitted) colours, respectively. (d,e) Computed electron band structures along the line used in the experimental study of the temperature evolution of the surface state spin split (inset inFig. 2d). Figure 3a shows the spatial extension of the Kohn-Sham eigenstate corresponding to the surface state at the point that has been found in the slab calculations. Clearly, the surface state is not strictly confined to the first atomic layer but extends over the first four layers up to the Eu ions. Figure 3b,c show the calculated bulk Fermi surface superimposed with that calculated for the slab in the PM and AFM phases. Respectively, the excellent agreement with the ARPES spectra depicted in Fig. 2a,b is evident. The bulk related calculations revealed for both phases a similar gap around the point, while the results of slab calculations nicely reproduce the discussed surface state, which lies inside this gap and clearly splits in the AFM phase. Note that a similar splitting is also obtained for the case that only the topmost Eu layer is ordered ferromagnetically while the bulk is already in the PM phase ( Supplementary Fig. 5a ). This provides strong evidence that the observed splitting in the ARPES experiment is indeed caused by the magnetic exchange interaction, lifting up the spin degeneracy of the surface state. Figure 3d,e present a similar cut, taken through the surface state parallel to – as in Fig. 2d , for the PM and AFM phases, respectively. Even quantitatively, the exchange splitting obtained from the calculations agrees well with our experimental findings (~138 versus ~150 meV). Both our findings, experimental and theoretical, show that the exchange splitting causes a strong anisotropy of the surface state with a difference of about 25 meV between the – and the - directions. Figure 3: Theoretical insight into surface and bulk related electrons in EuRh 2 Si 2. ( a ) Probability density distribution (projected on the ac plane) of the surface states at the point obtained for the PM phase, which is superimposed with the slab crystal structure used for band-structure calculations. ( b , c ) The computed and superimposed Fermi surfaces for bulk and slab calculations for the PM and AFM phases, respectively. Here, the diamond-shaped surface states lie in the huge gap (black) of the projected bulk bands (grey) around the point. For the PM and AFM phases the surface state is emphasized in green (unsplitted) and red-blue (splitted) colours, respectively. ( d , e ) Computed electron band structures along the line used in the experimental study of the temperature evolution of the surface state spin split (inset in Fig. 2d ). 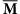Figure 4: Theoretically derived surface states at thepoint. Three-dimensional presentation of the surface state calculated for the AFM phase without (a) and with (b) consideration of spin–orbit effect. Close to thepoint the latter results in the opening of a gap connected with an avoided band crossing, and thus causes a change of the respective band spin character near the gap edges where these states are shown in grey. Full size image Figure 4a,b demonstrate the effect of spin–orbit interaction on the surface electron structure at the point for both the electron- and hole-like surface states. The inclusion of spin–orbit interaction practically does not modify the exchange interaction induced splitting. We can therefore safely claim that in general spin–orbit interaction only slightly influences the electron-like surface state splitting. However, spin–orbit interaction gets important in the immediate vicinity of the point: it produces a gap between the electron- and hole-like surface states with opposite spin in case of non-relativistic calculations ( Fig. 4b ), that is in excellent agreement with the experimental results ( Supplementary Figs 3,4 ). Figure 4: Theoretically derived surface states at the point. Three-dimensional presentation of the surface state calculated for the AFM phase without ( a ) and with ( b ) consideration of spin–orbit effect. Close to the point the latter results in the opening of a gap connected with an avoided band crossing, and thus causes a change of the respective band spin character near the gap edges where these states are shown in grey. Full size image Dressing band and origin of its splitting Interestingly, a closer look at the experimental and theoretical results reveals that a splitting in the AFM phase is not only observed for the prominent surface state but also for the sharp ‘dressing’ feature that surrounds it and is labelled ‘1’ in Fig. 2b . This band is reproduced in the bulk band-structure calculations and should, therefore, reflect bulk properties of the material. However, the splitting of the ‘dressing band’ reveals a similar temperature dependence as the surface state ( Fig. 2a ), which implies that (i) it is also related to magnetism and (ii) this spectral feature reflects to some extent the surface properties of the material. The latter may be understood taking into account the following. The wave functions of bulk states become modified at the surface leading in some cases to the formation of surface resonances characterized by an enhanced probability density in the near surface region. Since the ‘dressing band’ lies at the periphery of the gap at the point it is not unlikely that it may display surface resonance character. In contrast to the surface state, the splitting of the ‘dressing band’ seems linked to the symmetry breaking caused by the antiferromagnetic order. This is, for example, demonstrated by a calculation in which a superstructure is produced by replacing the divalent Eu atoms of every second Eu layer by trivalent Gd ions ( Supplementary Fig. 5b ). The results reveal a gap formation similar to that of pure EuRh 2 Si 2 in its AFM phase, although both the Eu and Gd ions were treated in the PM state. The fact that the gap persists, like the splitting of the surface state, well above the Néel temperature of the bulk indicates that the surface ordering is not restricted to the topmost Eu layer alone but extends over several Eu layers. Thus the temperature dependence of the dressing band’s splitting (see Fig. 2c ) is a further support for an interpretation in terms of a second-order phase transition of the near surface region differing from the bulk, instead of an order parameter fluctuation scenario. In summary, we have given clear evidence for a large exchange coupling of a Si-derived Shockley surface state to the outermost Eu layer that is located four atomic layers below the surface of the antiferromagnetic compound EuRh 2 Si 2 . The resulting exchange splitting provides direct information on the temperature-dependent magnetism in the discussed Eu layer and reveals an ordering temperature of 4 f moments close to the surface that is notably higher than the bulk T N . Our results suggest that the mechanism of formation of the surface ferromagnetism discovered in EuRh 2 Si 2 can be extended to other antiferromagnetic metallic or semiconducting compounds where surface states exist in an energy gap at the Fermi level. These spin-split surface states may induce magnetization in functional surface layers of topological insulators or/and Rashba-type surface systems deposited onto the antiferromagnetic material, thus opening an energy gap in the topological or Rashba-type surface states. Experiment ARPES studies were carried out at the Swiss Light Source (SIS X09LA instrument) as described in detail in Höppner et al . [13] The spectra were acquired using a Scienta R4000 electron energy analyser. The overall energy and angular resolutions were 10 meV and 0.1 degree, respectively. High quality single-crystalline samples of EuRh 2 Si 2 were cleaved in situ in ultra-high vacuum at a base pressure better than 8 × 10 −11 mbar. Surface regions terminated by a Si layer were selected by minimizing the Eu 4 f surface-related PE signal as the beam was scanned across the sample. For the Fermi surface measurements a new sample was cleaved at each temperature. The temperature-dependent measurements were performed always going from high to low temperatures in order to avoid fast sample aging. Resonant magnetic scattering experiments were carried out at the Eu L 3 edge using beamline P09, PETRA III, DESY. Theory The electron band structure of EuRh 2 Si 2 was calculated using DFT within the local density approximation in the parameterization of Perdew/Wang [21] in a full-potential local orbital basis [22] , with the scalar-relativistic approximation employed. The 4 f basis states of Eu have been fixed to the experimentally found occupation ( n 4f ≈7.0) using either an unpolarized, PM configuration or a local moment scenario of 7 μB per Eu atom and a ferromagnetic coupling within the Eu ab planes and AFM interaction along the c axis. This partial restriction of the basis set is called ‘open-core’ or ‘quasi-core’ approximation. The Si-terminated surface of the EuRh 2 Si 2 crystal has been simulated by a slab that breaks the translational invariance along the c axis and has at least seven successive Eu layers in the conventional unit cell. A detailed description can be found in the supplementary information of Höppner et al . [13] The k -mesh was set to (12 × 12 × 12) for the bulk and (12 × 12 × 1) for the slab calculations, respectively. We also performed DFT general gradient approximation (GGA) spin-polarized calculations employing the full-potential linearized augmented plane wave method as implemented in the FLEUR code [23] . In this case the surface was simulated by a 24-atomic layers slab with one side terminated by the Si atoms, and the other one by the Eu atoms. In the self-consistent calculations the k -mesh (8 × 8 × 1) and about 150 basis functions per atom were used and spin–orbit coupling was included as described by Li et al . [24] For a proper description of the Eu 4 f and Rh 4 d electrons, we apply the GGA+U method [25] in an implementation similar to that of Shick et al . [26] For the 4 f electrons of Eu, we used values of U =7.4 eV and J =1.1 eV, for the Rh 4 d electrons of U =3.4 eV and J =0.6 eV. These parameters were chosen to simulate the experimentally observed positions of the 4 f bands of Eu and 4 d bands of Rh. How to cite this article: Chikina, A. et al . Strong ferromagnetism at the surface of an antiferromagnet caused by buried magnetic moments. Nat. Commun. 5:3171 doi: 10.1038/ncomms4171 (2014).